Visualizing the atomic-scale electronic structure of the Ca2CuO2Cl2Mott insulator Although the mechanism of superconductivity in the cuprates remains elusive, it is generally agreed that at the heart of the problem is the physics of doped Mott insulators. A crucial step for solving the high temperature superconductivity puzzle is to elucidate the electronic structure of the parent compound and the behaviour of doped charge carriers. Here we use scanning tunnelling microscopy to investigate the atomic-scale electronic structure of the Ca 2 CuO 2 Cl 2 parent Mott insulator of the cuprates. The full electronic spectrum across the Mott–Hubbard gap is uncovered for the first time, which reveals the particle–hole symmetric and spatially uniform Hubbard bands. Defect-induced charge carriers are found to create broad in-gap electronic states that are strongly localized in space. We show that the electronic structure of pristine Mott insulator is consistent with the Zhang–Rice singlet model, but the peculiar features of the doped electronic states require further investigations. Soon after the discovery of high T C (critical temperature) superconductivity in the cuprates, it was realized that the superconducting phase lies in close proximity to an insulating state [1] . The cuprate parent compound has one unpaired electron per Cu site, and is predicted by band theory to be a half-filled metal. The strong onsite Coulomb repulsion, however, prohibits electron hopping between neighbouring sites and leads to a Mott insulator ground state with antiferromagnetic (AF) ordering. Charge carriers doped into the CuO 2 plane destroy the insulating phase and superconductivity emerges as the carrier density is sufficiently high. The main challenge in the quest for understanding high T C superconductivity is to describe the behaviour of the doped charge carriers in the presence of strong electron correlations [2] . A natural starting point for tackling this formidable task is to elucidate the electronic structure of the parent Mott insulator, and see how a single electron or hole behaves in the AF spin background. Despite extensive experimental studies on the parent and lightly doped Mott insulators, a comprehensive picture about their electronic structure is still lacking. Optical spectroscopy [3] and resonant inelastic X-ray spectroscopy [4] , [5] can probe the excitations across the Mott–Hubbard gap, but they cannot detect the ground-state electronic structure directly. Angle-resolved photoemission spectroscopy (ARPES) provides direct momentum ( k ) space structure of the occupied lower Hubbard band (LHB) [6] , [7] , but is unable to reach the empty states above the Fermi level ( E F ), leaving the upper Hubbard band (UHB) unexplored. The lack of complete spectroscopic information across the Mott–Hubbard gap makes it difficult to clarify how the high-energy spectral weight is transferred to the low-energy states near E F , upon which superconductivity emerges. Another vital piece of information that is still missing is the spatial characteristic of the Mott insulator electronic structure. As the Mott physics is dictated by onsite Coulomb repulsion, the real-space picture could be more relevant than the k -space picture, which has been extremely successful in describing weakly interacting electron systems. Especially, atomic-scale resolution becomes indispensible if we want to experimentally illustrate the electronic properties of a single charge doped into the AF background. Scanning tunnelling microscopy (STM) is an ideal spectroscopic technique for filling the aforementioned gaps in our understanding of doped Mott insulators. STM can directly map out the electronic states, both below and above E F , with the unique capability of atomic-scale spatial resolution. STM studies on high T C cuprates have revealed a variety of remarkable phenomena, including the impurity resonance [8] , [9] , checkerboard ordering [10] , [11] , [12] , [13] and phase incoherent Cooper pairing [14] , [15] . However, the parent Mott insulator phase has never been investigated by STM, most likely owing to the technical challenges associated with tunnelling into a good insulator. Here, we report the first STM study of the atomic-scale electronic structure of the Ca 2 CuO 2 Cl 2 (CCOC) parent Mott insulator of the cuprates. The full electronic spectrum across the Mott–Hubbard gap is uncovered by tunnelling spectroscopy, which reveals the particle–hole symmetric and spatially uniform Hubbard bands. Defect-induced charge carriers are found to create broad in-gap electronic states that are strongly localized in space. The electronic structure of the pristine Mott insulator is in good agreement with the single-band Zhang–Rice singlet (ZRS) model, but the peculiar features of the doped electronic states require further investigations. Topographical properties of the CCOC surface The oxychloride cuprate CCOC Mott insulator is chosen for its high crystal quality and excellent cleavage properties. 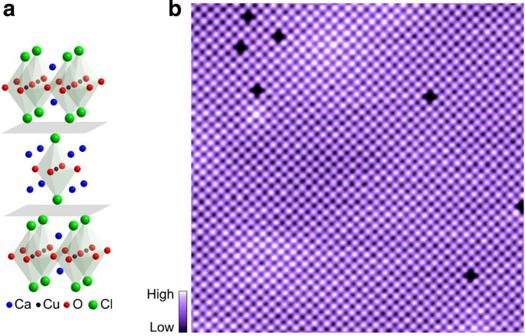Figure 1: Crystal structure and STM topography on CCOC. (a) Crystal structure of CCOC, which is similar to that of La2CuO4except that the LaO layer is replaced by CaCl layer. The crystal cleaves easily between two adjacent CaCl layers, as indicated by the grey planes, exposing the square lattice of Cl atoms. (b) Constant current topographical image (155 Å × 155 Å) of CCOC taken at bias voltageVs=−3.5 V and tunnelling currentIt=10 pA. Each cross-shaped dark site on the surface corresponds to a missing Cl defect. Figure 1a shows the schematic crystal structure of CCOC, which is similar to that of the prototypical parent compound La 2 CuO 4 . The crystal cleaves easily between two adjacent CaCl layers, exposing the Cl terminated surface. The CuO 2 plane lies at 2.73 Å below the surface and the Cu sites are directly underneath the exposed apical Cl atoms. The local electronic properties of hole-doped Ca 2-x Na x CuO 2 Cl 2 have been extensively studied by STM [13] , [16] , [17] , [18] . In this work, we report the first STM study of the pristine CCOC Mott insulator phase. Details about the sample growth and STM measurements are described in the Methods session and Supplementary Fig. S1 . Figure 1: Crystal structure and STM topography on CCOC. ( a ) Crystal structure of CCOC, which is similar to that of La 2 CuO 4 except that the LaO layer is replaced by CaCl layer. The crystal cleaves easily between two adjacent CaCl layers, as indicated by the grey planes, exposing the square lattice of Cl atoms. ( b ) Constant current topographical image (155 Å × 155 Å) of CCOC taken at bias voltage V s =−3.5 V and tunnelling current I t =10 pA. Each cross-shaped dark site on the surface corresponds to a missing Cl defect. Full size image Figure 1b displays a typical STM topography of cleaved CCOC taken at T =77 K with sample bias V s =−3.5 V and tunnelling current I t =10 pA, which reveals a large area of atomically flat terrace. The Cl atoms form a regular square lattice with lattice constant a ~3.9 Å, in agreement with the tetragonal unit cell of CCOC. The cross-shaped dark spots in the image correspond to the missing Cl defects (or Cl vacancies), which are created during the cleaving process. The inset of Fig. 2a displays the high-resolution STM image of a defect-free area, which has arguably the most ideal surface structure for the cuprates without the complications from structural supermodulations and electronic inhomogeneities. 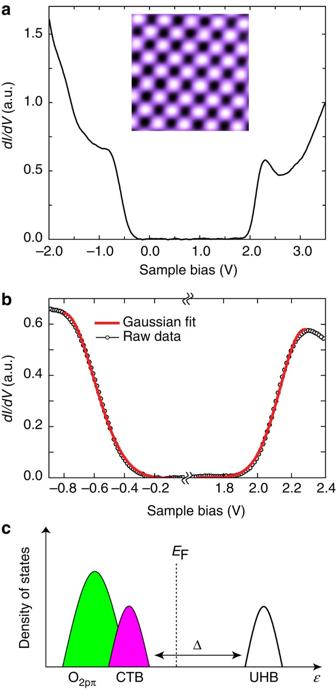Figure 2: Spectroscopy and electronic structure of pure CCOC. (a) Spatially averageddI/dVspectrum over a defect-free area of CCOC reveals the full electronic structure across the Mott gap. (Inset) High-resolution image (28 Å × 28 Å) of the area where the spectra are taken. (b) Closed-updI/dVcurves of the charge transfer band (CTB) and the upper Hubbard band (UHB). The red curves show the Gaussian fit to the data. (c) Schematic band structure of the pristine Mott insulator showing the UHB (unfilled), the CTB (pink) and the non-bonding O 2pπ band (green). Figure 2: Spectroscopy and electronic structure of pure CCOC. ( a ) Spatially averaged dI / dV spectrum over a defect-free area of CCOC reveals the full electronic structure across the Mott gap. (Inset) High-resolution image (28 Å × 28 Å) of the area where the spectra are taken. ( b ) Closed-up dI/dV curves of the charge transfer band (CTB) and the upper Hubbard band (UHB). The red curves show the Gaussian fit to the data. ( c ) Schematic band structure of the pristine Mott insulator showing the UHB (unfilled), the CTB (pink) and the non-bonding O 2 p π band (green). Full size image Electronic structure of pristine CCOC The local electronic structure of CCOC is probed by dI/dV (differential conductance) spectroscopy, which is approximately proportional to the electron density of state (DOS). Figure 2a displays the spatially averaged dI/dV curve obtained on the defect-free surface shown in the inset (the individual curves are displayed in the Supplementary Fig. S2 ). The full electronic spectrum across the Mott–Hubbard gap is directly uncovered for the first time. The occupied state dI/dV curve is very similar to the ARPES measured energy distribution curves of CCOC [6] , [19] , especially those along the (0, π) direction as discussed in Supplementary Fig. S3 and Supplementary Note 1 . As the parent cuprate is a charge transfer insulator with oxygen bands lying between the LHBs and UHBs [20] , the shoulder near V s =−0.8 V is ascribed to the charge transfer band (CTB) and the rapid increase for V s <−1.5 V is due to the non-bonding O 2 p π state [6] , [19] . The totally new feature revealed by Fig. 2a is the UHB above E F , which was an unexplored territory before this report. The simultaneous observation of CTB and UHB immediately reveals several key spectroscopic features of the Mott insulator. The effective Mott–Hubbard gap, or more precisely the charge transfer gap, can be directly measured to be Δ=2.2 eV. This value is very close to the 2.1 eV gap size obtained by optical reflectivity on parent CCOC [3] . The excellent agreement with the optical and ARPES results indicate that the tip-induced band bending, which may affect STM results on insulating materials, is negligible in our measurement. Shown in Fig. 2b are the zoom-in dI/dV curves of the CTB and UHB, which can fit well by using a broad Gaussian function rather than a sharper Lorentzian. Similar feature has been observed by previous ARPES measurements and interpreted as evidence for the breakdown of the coherent quasiparticle picture in Mott insulators [19] . The full-width at half-maximum for the CTB and UHB are Γ =0.47 and 0.34 eV, respectively, which are comparable to the bandwidth W =0.35 eV determined by the ARPES measured band dispersion [19] . The similar lineshape, bandwidth and peak DOS value of the CTB and UHB spectra demonstrate the approximate particle–hole symmetry across the charge transfer gap of the Mott insulator. The electronic structure of the Mott insulator phase is schematically illustrated in Fig. 2c . We next turn to the spatial distribution of the electronic structure, which is an issue of great importance to Mott insulator where the local Coulomb repulsion has a dominant role. As the lowest energy excitation of the charge transfer insulator is the removal of an electron from the occupied O 2 p orbital to the unoccupied Cu orbital [20] , naïvely it is expected that the unpaired hole will mainly reside on the anion ligands and electron on the cation d orbitals [21] . This picture implies that the relative weight of CTB and UHB may vary between the Cu and O sites. However, our atomically resolved dI/dV spectroscopy shown in Fig. 3 reveals that the entire electronic structure is highly uniform in space without significant difference between the Cu, O and Ca sites. This observation suggests that both the CTB and UHB of parent cuprate form extended states in space rather than keeping their local orbital characteristics. 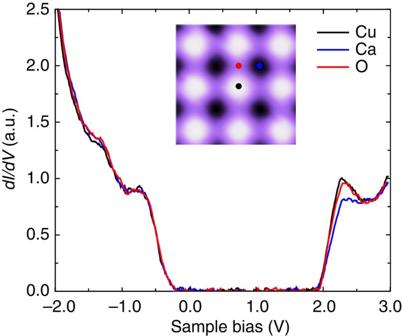Figure 3: Spatial distribution of the electronic structure in CCOC. The black, blue and red curves show the spatially resolveddI/dVspectra taken at the Cl (Cu), Ca and O sites of the CCOC surface, respectively. The setup conditions areVs=−3 V andIt=10 pA. There is no significant difference between the spectra, demonstrating spatially uniform electronic structures. (Inset) Closed-up topography of the pure CCOC surface. The black, blue and red dots indicate the locations where the corresponding spectra are taken. Figure 3: Spatial distribution of the electronic structure in CCOC. The black, blue and red curves show the spatially resolved dI/dV spectra taken at the Cl (Cu), Ca and O sites of the CCOC surface, respectively. The setup conditions are V s =−3 V and I t =10 pA. There is no significant difference between the spectra, demonstrating spatially uniform electronic structures. (Inset) Closed-up topography of the pure CCOC surface. The black, blue and red dots indicate the locations where the corresponding spectra are taken. Full size image Electronic states of doped charges Now that the electronic structure of pristine CCOC is well established, we are ready to investigate the electronic state created by an added charge. For this purpose, we take advantage of the defects that naturally occur in pristine CCOC. The most common defects on cleaved CCOC are the missing Cl atoms on the top surface, as revealed in Fig. 1b . As each Cl − ion strongly grasps an extra electron, a missing Cl effectively donates an electron into the CuO 2 plane. The red curve in Fig. 4a shows the dI/dV measured directly on the missing Cl site (or the exposed Cu site of the underneath CuO 2 plane) compared with that taken at a location far from the defect (black curve). The most dramatic spectroscopic feature caused by the doped electron is the emergence of a broad electronic state within the charge transfer gap near the edge of the UHB. Meanwhile, the peak of the UHB is completely suppressed, indicating the transfer of its spectral weight to the in-gap state. The CTB, in contrast, only shifts slightly, revealing a strong particle–hole asymmetry induced by the doped electron. As a consequence of the in-gap state, the local charge transfer gap at the defect centre is reduced to Δ=1.6 eV. The schematic electronic structure induced by the doped electron is drawn in Fig. 4b . 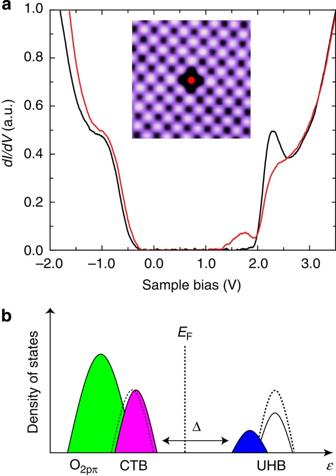Figure 4: Electronic structure of the missing Cl defect. (a) The red curve shows thedI/dVspectrum measured at the missing Cl defect centre and the black curve is taken at six lattice distances away from the defect. (Inset) High-resolution image (35 Å × 35 Å) around a missing Cl defect and the red dot indicates where the red curve is taken. (b) Schematic electronic structure at the defect centre: an in-gap state (blue) emerges near the edge of UHB owing to spectral weight transfer from the latter. The CTB is slightly shifted and the local gap amplitude is significantly reduced. Figure 4: Electronic structure of the missing Cl defect. ( a ) The red curve shows the dI/dV spectrum measured at the missing Cl defect centre and the black curve is taken at six lattice distances away from the defect. (Inset) High-resolution image (35 Å × 35 Å) around a missing Cl defect and the red dot indicates where the red curve is taken. ( b ) Schematic electronic structure at the defect centre: an in-gap state (blue) emerges near the edge of UHB owing to spectral weight transfer from the latter. The CTB is slightly shifted and the local gap amplitude is significantly reduced. Full size image The spatial distribution of the doped electronic state is another fundamental issue that STM is particularly suited for investigating. 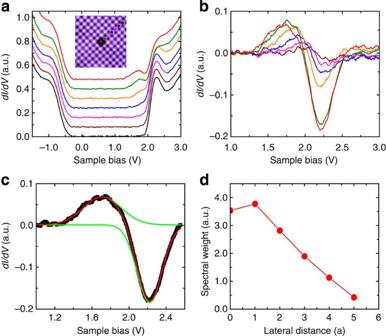Figure 5: Spatial distribution of the doped electronic state. (a) A series ofdI/dVspectra taken at locations away from the missing Cl defect centre along the Cu–O bond direction, as indicated in the inset by coloured dots. (b) Contribution of the doped electronic state to local electronic structure obtained by subtracting the backgrounddI/dV(acquired at six lattice distances away from the defect) from eachdI/dVspectrum ina. (c) The red curve inbcan fit well by two Gaussian terms and the spectral weight of the in-gap state can be estimated by the area enclosed by the Gaussian lineshape. (d) Spatial dependence of the in-gap state spectral weight, which decays rapidly with increasing lateral distance from the defect centre. Figure 5a shows a series of dI/dV spectra taken as the STM tip is positioned away from the defect centre along the Cu–O bond direction (inset of Fig. 5a ), which reveals the vanishing in-gap state accompanied by the emerging UHB peak. At a distance of six lattice constants from the defect centre, the dI/dV curve becomes similar to that of the pristine Mott insulator. By subtracting this background from the dI/dV curve at each location, the relative contribution of the defect state can be extracted. As shown in Fig. 5b , both the amplitude of the in-gap state and the suppression of UHB decrease systematically with increasing distance from the defect centre. Figure 5c shows that the profile can fit very well by using two Gaussian terms representing the created in-gap state and suppressed UHB, respectively (see Supplementary Fig. S4 for details). The spectral weight of the in-gap state can be roughly estimated by the area enclosed by the Gaussian fit ( Supplementary Note 2 ). Figure 5d summarizes the spatial evolution of the spectral weight, which loses half of its strength within a distance of three lattice sites, or merely 12 Å from the defect centre. The in-gap state is thus strongly localized in space, presumably owing to the frustrated motion of the doped charge in the AF background. Figure 5: Spatial distribution of the doped electronic state. ( a ) A series of dI/dV spectra taken at locations away from the missing Cl defect centre along the Cu–O bond direction, as indicated in the inset by coloured dots. ( b ) Contribution of the doped electronic state to local electronic structure obtained by subtracting the background dI/dV (acquired at six lattice distances away from the defect) from each dI/dV spectrum in a . ( c ) The red curve in b can fit well by two Gaussian terms and the spectral weight of the in-gap state can be estimated by the area enclosed by the Gaussian lineshape. ( d ) Spatial dependence of the in-gap state spectral weight, which decays rapidly with increasing lateral distance from the defect centre. Full size image Bias-dependent topography near the missing Cl defect reveals another highly unexpected feature. 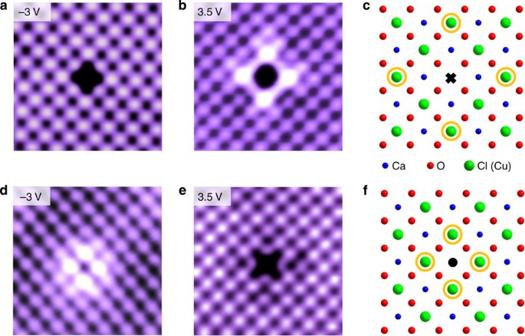Figure 6: Bias-dependent images around the defects. (a,b) Constant current images (35 Å × 35 Å) around a missing Cl defect taken at negative and positive biases, respectively. The positive-bias image shows four bright spots at the next-nearest-neighbour (NNN) Cu sites around the defect. (c) Schematic topview of the exposed surface showing the missing Cl defect (dark cross) and the NNN Cu sites (orange circles) with enhanced brightness at positive bias. (d,e) Constant current images (35 Å × 35 Å) around a Ca-site defect taken at the same biases asaandb. The most pronounced feature here is the strongly enhanced topographical intensity of the four nearest Cu sites in the negative-bias image. (f) Schematic structure showing the position of the Ca-site defect (dark dot) and the nearest-neighbour Cu sites (orange circles). Figure 6a shows the STM image taken at negative bias V s =−3.0 V, which probes the occupied state. Except for the missing Cl atom, there is no other pronounced spatial feature. Figure 6b displays the image taken at the same area with positive bias V s =3.5 V, which shows a dramatic spatial pattern where the four next-nearest-neighbour sites appear to be anomalously bright (illustrated in Fig. 6c ). The bias-dependent images further demonstrate the particle–hole asymmetry induced by the doped electron. Interestingly, similar patterns have been seen at Ni impurity in superconducting Bi 2 Sr 2 CaCu 2 O 8+δ , where the next-nearest-neighbour sites brighten up in the positive-bias DOS map [9] . It will be intriguing to find out if the spatial pattern of a doped electron in the Mott insulator is related to that of the Ni impurity states in superconducting cuprates. Figure 6: Bias-dependent images around the defects. ( a , b ) Constant current images (35 Å × 35 Å) around a missing Cl defect taken at negative and positive biases, respectively. The positive-bias image shows four bright spots at the next-nearest-neighbour (NNN) Cu sites around the defect. ( c ) Schematic topview of the exposed surface showing the missing Cl defect (dark cross) and the NNN Cu sites (orange circles) with enhanced brightness at positive bias. ( d , e ) Constant current images (35 Å × 35 Å) around a Ca-site defect taken at the same biases as a and b . The most pronounced feature here is the strongly enhanced topographical intensity of the four nearest Cu sites in the negative-bias image. ( f ) Schematic structure showing the position of the Ca-site defect (dark dot) and the nearest-neighbour Cu sites (orange circles). Full size image Besides the well-defined missing Cl defect on the surface, there exists another type of defect that occurs in the bulk of CCOC. Figure 6d show the topographical images around such a defect at negative and positive biases, respectively. The images exhibit totally different bias dependence as compared with that of the missing Cl defect. The four nearest-neighbour Cu sites around the defect centre become anomalously bright at negative bias, while at positive bias they are slightly suppressed. In both images, the surface Cl layer retains the perfect crystalline order, and the defect is located at the centre of the four-Cl plaquette in the underneath layer, which corresponds to the Ca site as illustrated in Fig. 6f . 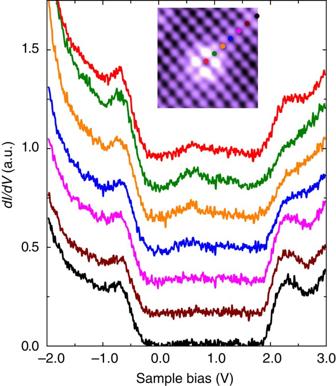Figure 7: Spatially resolved electronic structure near the Ca-site defect. dI/dVspectra taken at locations away from the Ca-site defect centre along the Cu–O bond direction, as indicated in the inset image (35 Å × 35 Å) by coloured dots. A broad in-gap state emerges at the defect site. It decays rapidly when moving away from the defect centre and vanishes beyond three lattice sites. Figure 7 displays the dI/dV spectra around the Ca-site defect at the locations marked by the dots in the inset. Right at the defect centre (the red curve), the spectrum also shows a broad in-gap state. It lies close to the lower edge of the charge transfer gap, rather than the upper gap edge as the missing Cl defect. Nevertheless, the electron DOS at E F is still zero, consistent with an insulating state. The in-gap state intensity drops rapidly with increasing distance from the defect and becomes negligibly small beyond three lattice constants from the defect centre. Therefore, the in-gap state is also strongly localized in space. Figure 7: Spatially resolved electronic structure near the Ca-site defect. dI/dV spectra taken at locations away from the Ca-site defect centre along the Cu–O bond direction, as indicated in the inset image (35 Å × 35 Å) by coloured dots. A broad in-gap state emerges at the defect site. It decays rapidly when moving away from the defect centre and vanishes beyond three lattice sites. Full size image The exact nature of the Ca-site defects is unknown at the current stage, but most likely they donate holes into the Mott insulator. From crystal chemistry point of view, there are two common types of Ca-site defects in CCOC: Ca vacancies due to the high growth temperature and Na substitution of Ca induced by the trace amount of Na impurities during the crystal growth process. Both types of defects are hole donors. The former one donates two holes and the later one donates one hole. CCOC with sufficient amount of Ca vacancies [22] or Na dopings [23] have been found to be hole-type superconductors. Furthermore, our STM results show that both the bias dependence of topography and the position of in-gap state on the Ca-site defect are opposite to that of the electron–donor Cl vacancy. As both features are closely related to the doped charge in the Mott insulator, they are also indicative of local hole doping. We note that these are only indirect evidences. To definitively find out the chemical nature of the Ca-site defect, future STM studies on CCOC with controlled amount of Ca vacancies or Na dopants are needed. The properties of parent and lightly doped cuprates are crucial to the mechanism of high T C superconductivity and have attracted tremendous theoretical interests [2] . It was first proposed by Anderson that the essential physics is contained in the half-filled Hubbard model [1] : Here, t is the hopping integral between nearest-neighbour sites and U is the onsite Coulomb repulsion. In the large U limit as in the cuprates, the Hubbard model is transformed into the t-J model, where J =4 t 2 / U is the superexchange energy. As the two-dimensional Hubbard or t-J models have yet to be solved exactly, various approximation schemes or numerical methods have been employed. The STM results shown here provide unprecedented real-space information and full electronic spectrum that can help discriminate the different models. A major theoretical debate is whether a single-band model is a valid low-energy model for the cuprates [24] . The charge transfer nature of the parent insulator suggests that a three band model involving two O bands and one Cu band might be more appropriate. However, it was proposed that the lowest hole-doped state, namely the CTB, can be represented by a single ZRS band [25] , in which the doped hole residing resonantly in the four planar O sites form a singlet with the central Cu 2+ ion. There are two specific predictions in the ZRS picture. First, the Mott insulator phase has particle–hole symmetry and second, the ZRS can move freely through the Cu 2+ lattice and thus should distribute uniformly in space. Our STM results show that undoped CCOC indeed has a nearly particle–hole symmetric and spatially uniform electronic structure, apparently supporting the single-band ZRS model. More quantitatively, the bandwidth of the CTB and UHB estimated from the Gaussian fit is in the order of 3 J ( J =0.13 eV in cuprate), which is also consistent with the calculation based on the single-band t-J model [26] . The electronic state induced by a doped charge has also been investigated extensively by theory [27] . A key issue here is whether the main effect of charge doping is the shift of E F or the emergence of new states or both. In both the missing Cl and Ca-site defects in CCOC, our STM results demonstrate that a new electronic state is always induced within the charge transfer gap, whereas the position of the Fermi level remains nearly unchanged. We next present a more careful examination of the doped electronic state. In the well-defined missing Cl defect, we find that the doped electron induces an in-gap state near the upper gap edge with its spectral weight mainly transferred from the UHB. The CTB has negligible contribution to the spectral weight transfer. This is inconsistent with the existing theory for electron-doped charge transfer insulators, in which both the CTB and UHB are expected to transfer spectral weight to the in-gap state [28] . We note that the electron donated by a surface defect studied here may not be an ideal situation owing to the change of local bonding situation and the existence of a defect potential, which may affect both the electronic spectrum and its spatial distributions. The quantitative explanation of these features may require a more sophisticated theoretical treatment like that for the impurity state in superconducting cuprates [29] . For the Ca-site defect, the in-gap state lies near the lower gap edge with vanishing DOS at E F . These features are in rough agreement with the calculated DOS for Mott insulator doped with few holes [30] . As the nature of the defect is still unknown, we will not elaborate on the theoretical implications of the STM results on the Ca-site defect. Another highly controversial issue regarding doped Mott insulator is whether a doped charge behaves like a coherent quasiparticle. Our STM results on both types of defects demonstrate that the in-gap state has a broad energy distribution and is strongly localized in space. Both features suggest that the doped charge does not behave like a coherent quasiparticle, presumably owing to the strong correlation effect. Indeed, recent theoretical studies show that a single charge doped into the AF Mott insulator is self-localized with vanishing quasiparticle weight [31] , [32] . The atomic-scale STM studies reported here demonstrate that the gross features of the electronic structure of pristine CCOC are consistent with the ZRS model. Although the quantitative in-gap state spectrum and its peculiar spatial variations cannot be explained readily by existing theory, we show that the emergence of a spatially localized in-gap state is generic for doped Mott insulators. In particular, the surface electron–donor defect represents a well-defined benchmark problem for testing the validity of various many body theories for doped Mott insulators. More importantly, our experiments establish a solid starting point for tackling the high T C problem. The obvious next step is to apply the atomic-scale large-bias spectroscopy to cuprates with increased dopings, which may elucidate how the Mottness eventually leads to high T C superconductivity. Sample growth The single crystals of Ca 2 CuO 2 Cl 2 (CCOC) are grown by the flux method as described elsewhere [23] . The powders of CaO and CuCl 2 are mixed with a molar ratio of 2:1 and put into an alumina crucible. The mixed powder is heated at 1,053 K for 24 h with intermediate grindings. After that, the CCOC precursor is heated to 1,053 K at a ramp rate of 60 K h −1 and kept at this temperature for 5 h. It is then heated to 1,203 K at a ramp rate of 60 K h −1 and kept at that temperature for 10 h. In the end, it is cooled down to room temperature at a ramp rate of 60 K h −1 . Single crystals with typical size of 2 mm × 2 mm × 0.1 mm can be harvested by cleaving the as-grown bulks. STM measurements The STM experiments are performed with a cryogenic variable temperature ultrahigh vacuum STM system. The CCOC crystal is cleaved in situ at T =77 K and then transferred immediately into the STM sample stage. To make tunnelling into the insulating CCOC possible, the STM experiments have to be performed at relative high temperature so that the sample has finite conductivity. At T =5 K, the STM tip will crash into the sample because the sample is so insulating that no tunnelling current can be detected. Therefore, all STM results reported in this paper are acquired at T =77 K. In addition to that, the sample bias voltage has to be set beyond the charge transfer gap so that there is finite DOS in the sample. The typical setup parameters are sample bias V s =±3 V and tunnelling current I t =2–10 pA. The STM topography is taken in the constant current mode, and the dI/dV spectra on CCOC are collected using a standard lock-in technique with modulation frequency f =423 Hz. To ensure the reliability of our high-energy tunnelling spectroscopy, we have developed a routine for STM tip treatment and calibration. The tip has to be stable under high biases, and its electronic DOS should be relatively featureless over a wide energy window. We use electrochemically etched polycrystalline tungsten tip for all the measurement. Before the STM experiments on CCOC, the tip is first treated by in situ high voltage e-beam sputtering, which is very efficient for cleaning and sharpening the tip. We then use the tip to approach an atomically clean crystalline Au(111) surface prepared in situ by repeated Ne ion sputtering and high temperature annealing. By taking topographical scans and spectroscopic measurements on clean Au(111) surface, we could check if the tip shape and spectrum are ideal. If necessary, further tip treatment can be done by field emission process or controlled gentle crash into the Au(111) crystal. Typical calibration data are shown in Supplementary Fig. S1 , where both the topography and spectroscopy indicate that the tip is clean and stable. High-quality large-bias, high temperature STM results can usually be obtained with such a tungsten tip. How to cite this article: Ye, C. et al. Visualizing the atomic-scale electronic structure of the Ca 2 CuO 2 Cl 2 Mott insulator. Nat. Commun. 4:1365 doi: 10.1038/ncomms2369 (2013).